Growth-regulatingMycobacterium tuberculosisVapC-mt4 toxin is an isoacceptor-specific tRNase Toxin–antitoxin (TA) systems are implicated in the downregulation of bacterial cell growth associated with stress survival and latent tuberculosis infection, yet the activities and intracellular targets of these TA toxins are largely uncharacterized. Here, we use a specialized RNA-seq approach to identify targets of a Mycobacterium tuberculosis VapC TA toxin, VapC-mt4 (also known as VapC4), which have eluded detection using conventional approaches. Distinct from the one other characterized VapC toxin in M. tuberculosis that cuts 23S rRNA at the sarcin–ricin loop, VapC-mt4 selectively targets three of the 45 M. tuberculosis tRNAs (tRNA Ala2 , tRNA Ser26 and tRNA Ser24 ) for cleavage at, or adjacent to, their anticodons, resulting in the generation of tRNA halves. While tRNA cleavage is sometimes enlisted as a bacterial host defense mechanism, VapC-mt4 instead alters specific tRNAs to inhibit translation and modulate growth. This stress-linked activity of VapC-mt4 mirrors basic features of eukaryotic tRNases that also generate tRNA halves and inhibit translation in response to stress. M ycobacterium tuberculosis has adapted to survive a wide range of assaults—from our immune response to antimicrobial therapeutics—intended to eradicate the organism. However, we lack a full understanding of the molecular switches that enable M. tuberculosis to endure these stresses, to slow replication or to become dormant as a latent tuberculosis infection. Emerging studies on the molecular underpinnings of stress survival in Escherichia coli generally point to a major role for chromosomal toxin–antitoxin (TA) systems, which are operons comprising adjacent genes encoding two small ( ∼ 10 kDa) proteins—a toxin and its cognate antitoxin that inhibits toxin activity in the TA protein–protein complex. The first described chromosomal TA system was E. coli mazEF , which was found to be induced by stress [1] , [2] . E. coli mazEF causes growth arrest and eventually cell death [1] , [2] . These studies and those on other TA systems in E. coli are consistent with a general role for TA systems in cell survival during periods of stress [3] . Observations in M. tuberculosis suggest that TA systems are also important for stress survival in this organism. Several TA loci in M. tuberculosis are induced during heat shock [4] , hypoxia [5] , [6] , DNA damage [7] , nutrient starvation [8] , macrophage infection [5] , [9] , [10] and antibiotic treatment [11] , [12] . Most recently, RNA-seq analysis of M. tuberculosis cells subjected to starvation revealed that the majority of TA systems, 75%, were upregulated to some degree with 25% upregulated twofold or higher [13] . The M. tuberculosis genome contains an estimated 48 members [5] , [14] of the VapBC (virulence-associated protein) family, the highest number of VapBC TA systems among free-living bacteria. VapC toxins are characterized by the presence of a PIN (PilT amino-terminal) domain. The 48 M. tuberculosis VapC toxins all share protein sequence similarity and possess a PIN domain containing a conserved quartet of acidic residues and a fifth invariant serine or threonine residue, which are responsible for coordinating divalent cation(s) in the catalytic centre [15] . The presence of a PIN domain suggests a role for the VapC toxins as ribonucleases, yet the body of literature on the enzymatic activity of VapC toxins has been inconsistent and contradictory. In our opinion, the most consistent data are derived from five recent reports. First, the solitary VapC toxin in Shigella or Salmonella cleaves tRNA fMet at a single, identical site in the anticodon stem loop (ASL) [16] . The solitary VapC in the spirochaete Leptospira interrogans also cleaves tRNA fMet (ref. 17 ). Second, the VapC from M. smegmatis cleaves synthetic ssRNAs at a short consensus sequence with some dependence on secondary structure [18] . In vivo , this VapC cleaves mRNA transcripts to downregulate M. smegmatis glycerol uptake and metabolism [18] . Third, we determined that a representative M. tuberculosis VapC toxin, VapC-mt4 (Rv0595c, also known as VapC4), recognizes ACGC or AC(A/U)GC in RNA [19] . Fourth, another M. tuberculosis VapC toxin, VapC20 (VapC-mt20 using our convention), cleaves at the highly conserved sarcin–ricin loop of 23S rRNA in intact ribosomes only, with some sequence specificity [20] . A detailed understanding of the properties of the 48 VapC paralogs is essential for the interpretation of their physiological role in M. tuberculosis and other pathogens. In this study, we identify the primary target of VapC-mt4 using a specialized RNA-seq approach. Distinct from all other VapC toxins, and TA toxins in general, VapC-mt4 arrests growth by translation inhibition resulting from selectively targeting three of the 45 tRNAs present in M. tuberculosis for cleavage at a single site in their anticodon loop. This highly selective tRNA substrate discrimination is contingent on recognition of the consensus sequence in an appropriate structural context. In agreement, VapC-mt4-tRNA-simulated docking experiments place the toxin active site in proximity to the cleavage site in the tRNA anticodon loop. Overall, these studies bring to light a common theme between the role of VapC-mt4 in this pathogen and stress responses in eukaryotic cells that also engage cleaved tRNAs in unconventional roles. RNA-seq reveals VapC-mt4 cleaves specific tRNA isoacceptors Our earlier study of VapC-mt4 revealed that this toxin inhibits translation and cleaves RNA at a consensus sequence of ACGC or AC(U/A)GC and that the GC sequence within this motif is essential for cleavage [19] . However, we were unable to clearly identify a primary target for this toxin. Although our data suggested that tRNA(s) may be the primary targets for M. tuberculosis VapC-mt4, we were unable to establish this connection using a battery of conventional biochemical, genetic and molecular biological approaches [19] . To overcome this roadblock, we used a specialized RNA-seq method we recently developed to identify RNA targets of endoribonucleolytic toxins [21] . This RNA-seq method was designed to differentially detect RNA cleavage products that carry a 5′-hydroxyl (OH) or a 5′-monophosphate (P). Bacterial transcripts possess a 5′-triphosphate (mRNAs), 5′-monophosphate (rRNAs and tRNAs) or 5′-hydroxyl (noncoding RNA intermediates and products cleaved by certain endoribonucleolytic toxins such as MazF or RNases such as RNase A and T1 (ref. 22 )). Another important feature of this RNA-seq method is its use of E. coli as a surrogate host, which unlike M. tuberculosis , does not contain a 5′-to-3′ exoribonuclease. Thus, the 5′ ends generated by VapC-mt4 cleavage can be readily detected because they will be stable. Using matrix-assisted laser desorption/ionization time-of-flight mass spectrometry, McKenzie et al. [23] reported that VapC toxins generate a 5′-P cleavage product. However, Winther and Gerdes suggested that the ends were instead marked with a 5′-OH because the 5′ terminus of the 3′ VapC RNA product could be phosphorylated without a prior dephosphorylation step [16] . Therefore, we constructed both 5′-P and 5′-OH cDNA libraries from RNA harvested from exponentially growing E. coli cells expressing VapC-mt4 from an arabinose-inducible vector. We did not identify any RNAs enriched by 10-fold or more in the 5′-P library relative to the uninduced control. In contrast, in the 5′-OH library, a cleavage product derived from three identical tRNAs—tRNA Ala2 , tRNA Ala41 and tRNA Ala58 —exhibited a 171-fold increase in transcript abundance, relative to the uninduced control ( Fig. 1a ). For simplicity, we will refer to these three identical tRNAs as tRNA Ala2 from this point forward (numbering based on the GtRNAdb Genomic tRNA Database [24] ). The sequence immediately upstream and downstream of the 5′ end of the cleavage site, A 37 C 38 ↓G 39 C 40 (where↓indicates the position of cleavage) was a 100% match to the recognition sequence deduced from our published in vivo and in vitro primer extension experiments [19] . Generation of the putative tRNA Ala2 cleavage product was specific to VapC-mt4 induction; we did not detect any other tRNA fragment that displayed more than a 10-fold increase in abundance in the comparison of 5′-OH libraries derived from VapC-mt4-induced cells relative to uninduced cells ( Supplementary Fig. 1 ). 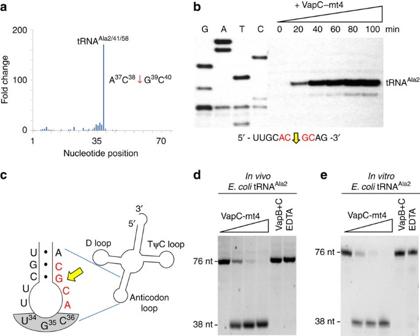Figure 1: VapC-mt4 Cleaves tRNAAla2inE. coli. (a) Histogram representing the fold change in 5′-OH ends observed along the length of the tRNAAla2upon comparison of cells with VapC-mt4 to those without VapC-mt4. The sequence surrounding the site of cleavage in tRNAAla2is shown on the right; red arrow denotes position of cleavage. (b) Primer extension analysis with totalE. coliRNA following the induction of VapC-mt4 for the times indicated. The RNA sequence (ACGC consensus in red) and positions of cleavage (yellow arrow) shown below the gel image. G, A, T and C lanes correspond to DNA-sequencing ladders using the same primer and a tRNAAla2DNA template. The major primer extension band migrates between the G and T residues in the sequencing ladder instead of aligning exactly to the G residue. We attribute this to the repeatable aberrant migration of the sequencing ladder below this tRNA sequence. (c) Illustration of the RNA-seq cleavage site in the tRNAAla2ASL, yellow arrow; ACGC consensus sequence in red, anticodon shaded in grey. (d,e) Cleavage assay within vivopurified tRNAAla2(d) orin vitro-synthesized tRNAAla2(e) and increasing amounts of VapC-mt4 (ratios of toxin to RNA were 0:1, 1.25:1, 2.5:1 and 5:1). Control reactions on the right contained the highest concentration of VapC-mt4 preincubated with VapB antitoxin or EDTA before addition of the respective tRNAs. Reactions were incubated at 37 °C for 3 h. Sizes of full-length and cleaved tRNA products on the left. Complete gel images for (b,d,e) are shown inSupplementary Fig. 2. Figure 1: VapC-mt4 Cleaves tRNA Ala2 in E. coli . ( a ) Histogram representing the fold change in 5′-OH ends observed along the length of the tRNA Ala2 upon comparison of cells with VapC-mt4 to those without VapC-mt4. The sequence surrounding the site of cleavage in tRNA Ala2 is shown on the right; red arrow denotes position of cleavage. ( b ) Primer extension analysis with total E. coli RNA following the induction of VapC-mt4 for the times indicated. The RNA sequence (ACGC consensus in red) and positions of cleavage (yellow arrow) shown below the gel image. G, A, T and C lanes correspond to DNA-sequencing ladders using the same primer and a tRNA Ala2 DNA template. The major primer extension band migrates between the G and T residues in the sequencing ladder instead of aligning exactly to the G residue. We attribute this to the repeatable aberrant migration of the sequencing ladder below this tRNA sequence. ( c ) Illustration of the RNA-seq cleavage site in the tRNA Ala2 ASL, yellow arrow; ACGC consensus sequence in red, anticodon shaded in grey. ( d,e ) Cleavage assay with in vivo purified tRNA Ala2 ( d ) or in vitro -synthesized tRNA Ala2 ( e ) and increasing amounts of VapC-mt4 (ratios of toxin to RNA were 0:1, 1.25:1, 2.5:1 and 5:1). Control reactions on the right contained the highest concentration of VapC-mt4 preincubated with VapB antitoxin or EDTA before addition of the respective tRNAs. Reactions were incubated at 37 °C for 3 h. Sizes of full-length and cleaved tRNA products on the left. Complete gel images for ( b , d , e ) are shown in Supplementary Fig. 2 . Full size image Validation of VapC-mt4 specificity for E. coli tRNA Ala2 We proceeded to confirm our RNA-seq result (plotted in Fig. 1a ) suggesting that tRNA Ala2 is a major target for cleavage by VapC-mt4 using two approaches. In the first approach, we performed primer extension on the RNA samples from E. coli cells 0, 20, 40, 60, 80 and 100 min after induction. A strong cleavage product accumulated with time at the same site in tRNA Ala2 identified by RNA-seq ( Fig. 1b and Supplementary Fig. 2 ). The validated RNA-seq cleavage site mapped to the junction of the stem and loop in the ASL ( Fig. 1c ). For our second approach, we purified tRNA Ala2 from total E. coli RNA using a biotinylated oligonucleotide complementary to a sequence in the ASL unique to this isoacceptor. Incubation of pure VapC-mt4 with this tRNA Ala2 led to complete cleavage with increasing toxin concentration, generating products consistent with cleavage at the A 37 C 38 ↓G 39 C 40 site in the ASL identified by RNA-seq and primer extension ( Fig. 1d ). Cleavage was abolished when VapC-mt4 was preincubated with its cognate antitoxin VapB-mt4 and when EDTA was added to the reaction to chelate Mg 2+ ( Fig. 1d ). Although none of the bases comprising the ACGC sequence in E. coli tRNA Ala2 cleaved by VapC-mt4 are modified, modifications in proximal bases may enhance cleavage (for example, there is a 7-methylguanosine at position 46 of tRNA Ala2 ). To address this, we compared the efficiency of cleavage of tRNA Ala2 produced in vivo containing modified bases ( Fig. 1d ) with that synthesized in vitro lacking modified bases ( Fig. 1e ). There was no difference in the efficiency of cleavage between the two versions of tRNA Ala2 , indicating that base modifications in this tRNA are not required for VapC-mt4 cleavage. Cleavage by VapC-mt4 was also specific for tRNA Ala2 since non-ACGC-containing tRNAs (tRNA fMet (ref. 19 )) or other ACGC-containing tRNAs (for example, tRNA Asp3 ) subjected to the same reaction as Fig. 1e were not cleaved. Therefore, our RNA-seq approach was a valid predictor of the VapC-mt4 RNA target and site of cleavage in E. coli cells because tRNA Ala2 , but no other tRNA ( Supplementary Fig. 1 ), was cleaved at the same site both in vivo and in vitro . VapC-mt4 cleaves three M. tuberculosis tRNAs within the ASL Our RNA-seq analysis suggested that VapC-mt4 generally targets tRNA and not rRNA as recently reported for VapC-mt20 (ref. 20 ). Since VapC-mt4 cleavage of tRNA Ala2 did not require base modifications ( Fig. 1d,e ), we used synthetic tRNAs to test toxin specificity for all M. tuberculosis tRNAs containing a consensus sequences. ACGC was the predominant in vivo cleavage site identified by our earlier in vivo primer extension experiments [19] and was also represented in the highest ranking RNA-seq target, tRNA Ala2 . We surveyed all 45 tRNAs in M. tuberculosis (all but three—two tRNA Met and one tRNA fMet —have unique anticodons) and identified 13 distinct tRNAs with ACGC or the related ACAGC or ACUGC cleavage consensus sequences [19] . We synthesized each of these 13 M. tuberculosis tRNAs and subjected them to the same VapC-mt4 in vitro cleavage assay used in Fig. 1d,e . VapC-mt4 exhibited a strong preference for three of the 13 tRNAs (that is, complete cleavage of full-length tRNA), tRNA Ala2 ( Fig. 2a ), tRNA Ser26 ( Fig. 2b ) and tRNA Ser24 ( Fig. 2c ). Preincubation of VapC-mt4 with either its cognate antitoxin VapB-mt4 or EDTA prevented tRNA cleavage. tRNA Glu33 , representative of the 10 tRNAs that were either weakly cut or not cut at all, is shown in Fig. 2d . The entire set of 10 consensus site-containing tRNAs that were tested for cleavage and not classified as a VapC-mt4 target is shown in Supplementary Fig. 3 ). Therefore, VapC-mt4 efficiently cleaved only 3 of 13 M. tuberculosis tRNAs harbouring the cleavage consensus sequence. Although VapC-mt4 cleaved tRNAs with the same name (tRNA Ala2 from E. coli and M. tuberculosis ), these tRNAs are not identical (71% identical overall among their 76 nts). However, there is high identity in the most relevant portion of these two tRNAs: the anticodon loop. The first 7 nts (which includes the anticodon) of the 9 nt loop are identical. 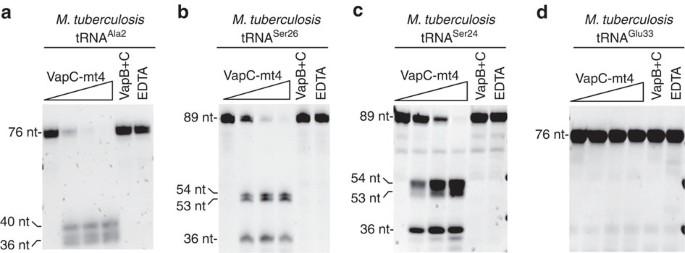Figure 2: VapC-mt4 targets a specific subset of tRNAs inM. tuberculosis. (a–c)In vitroVapC-mt4 cleavage assays showing the three tRNAs from among the 13 consensus-containingM. tuberculosistRNAs tested that are cleaved to completion: tRNAAla2(a), tRNASer26(b) and tRNASer24(c). (d) tRNAGlu33is shown as a representative example of a tRNA not cut by VapC-mt4 even though it contains the cleavage consensus sequence.In vitro-synthesized tRNAs were incubated with increasing amounts of VapC-mt4 (ratios of toxin to RNA were 0:1, 1.25:1, 2.5:1, and 5:1). Control reactions on the right contained the highest concentration of VapC-mt4 preincubated with VapB antitoxin or EDTA before addition of the respective tRNAs. Reactions were incubated at 37 °C for 3 h. Sizes of full-length and cleaved tRNA products are indicated on the left. Note that in some cases extra bands are visible for the cleavage products because the T7 RNA polymerase used to synthesize the tRNAs frequently leads to 3′ end heterogeneity (usually ±1 nt)61,62. Complete gel images fora–care shown inSupplementary Fig. 3. Complete gel images fordalong with full gels images of all 10 tRNAs that were weakly cut or not cut at all are shown inSupplementary Fig. 4. Figure 2: VapC-mt4 targets a specific subset of tRNAs in M. tuberculosis . ( a – c ) In vitro VapC-mt4 cleavage assays showing the three tRNAs from among the 13 consensus-containing M. tuberculosis tRNAs tested that are cleaved to completion: tRNA Ala2 ( a ), tRNA Ser26 ( b ) and tRNA Ser24 ( c ). ( d ) tRNA Glu33 is shown as a representative example of a tRNA not cut by VapC-mt4 even though it contains the cleavage consensus sequence. In vitro -synthesized tRNAs were incubated with increasing amounts of VapC-mt4 (ratios of toxin to RNA were 0:1, 1.25:1, 2.5:1, and 5:1). Control reactions on the right contained the highest concentration of VapC-mt4 preincubated with VapB antitoxin or EDTA before addition of the respective tRNAs. Reactions were incubated at 37 °C for 3 h. Sizes of full-length and cleaved tRNA products are indicated on the left. Note that in some cases extra bands are visible for the cleavage products because the T7 RNA polymerase used to synthesize the tRNAs frequently leads to 3′ end heterogeneity (usually ±1 nt) [61] , [62] . Complete gel images for a – c are shown in Supplementary Fig. 3 . Complete gel images for d along with full gels images of all 10 tRNAs that were weakly cut or not cut at all are shown in Supplementary Fig. 4 . Full size image We then used primer extension to identify the position of VapC-mt4 cleavage in the synthetic tRNAs shown in Fig. 2 . Using this approach, all three tRNA cleavage sites mapped within the anticodon loop ( Fig. 3a,c,e and Supplementary Fig. 4 ). Finally, we confirmed that VapC-mt4 efficiently cleaves tRNAs from M. tuberculosis cells. We isolated total RNA from M. tuberculosis and incubated it with VapC-mt4 alone or VapC-mt4 preincubated with its cognate antitoxin VapB-mt4 as a control. We then performed northern analysis with an isoacceptor-specific oligonucleotide complementary to the ASL for tRNA Ser26 or tRNA Ser24 ( Fig. 4a,b ); we also performed a similar experiment for E. coli tRNA Ala2 as a control ( Fig. 4c ). Addition of VapC-mt4 resulted in the loss of hybridization, indicating that the respective tRNAs were cleaved ( Fig. 4a–c ). In the case of M. tuberculosis tRNA Ala2 , sequence similarity among alanine isoacceptor tRNAs was too high to enable selective hybridization for only tRNA Ala2 . In summary, VapC-mt4 cleaves three M. tuberculosis tRNAs within their anticodons (tRNA Ser24 and tRNA Ser26 ; when referring to both of these tRNAs they will subsequently be called tRNA Ser24/6 ) or immediately 3′ of the anticodon (tRNA Ala2 ). As with E. coli tRNA Ala2 , this cleavage appears to be efficient in the presence or absence of tRNA modifications. 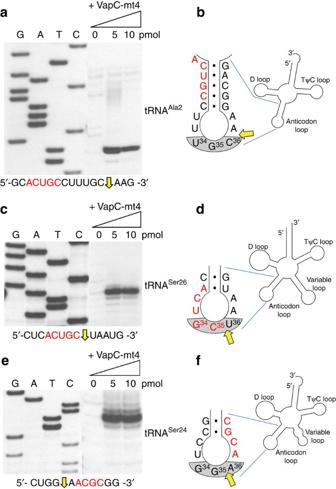Figure 3: VapC-mt4 cleaves threeM. tuberculosistRNAs near consensus sequences. (a–f) Primer extension analysis within vitro-synthesizedM. tuberculosistRNAAla2(a,b), tRNASer26(c,d) and tRNASer24(e,f). The RNA sequence (ACGC or ACUGC consensus in red) and positions of cleavage (yellow arrow) shown below gel images in left panels. G, A, T and C lanes correspond to DNA-sequencing ladders using the same primer and matched tRNA DNA template as the corresponding primer extension. To the right of each primer extension are illustrations highlighting the cleavage site (yellow arrow) relative to the consensus sequence (red) and anticodon (grey shaded). tRNAs were incubated with increasing amounts of VapC-mt4 (ratios of toxin to RNA were 0:1, 2.5:1 and 5:1) for 3 h at 37 °C. Convention when numbering tRNA bases dictates that the anticodon is designated as numbered positions 34–36. This convention is followed inb,d,f. Note, however, that for tRNASer26(d) and tRNASer24(f) the actual base numbers for the anticodon are 35–37. Complete gel images are shown inSupplementary Fig. 5. Figure 3: VapC-mt4 cleaves three M. tuberculosis tRNAs near consensus sequences. ( a–f ) Primer extension analysis with in vitro -synthesized M. tuberculosis tRNA Ala2 ( a,b ), tRNA Ser26 ( c,d ) and tRNA Ser24 ( e,f ). The RNA sequence (ACGC or ACUGC consensus in red) and positions of cleavage (yellow arrow) shown below gel images in left panels. G, A, T and C lanes correspond to DNA-sequencing ladders using the same primer and matched tRNA DNA template as the corresponding primer extension. To the right of each primer extension are illustrations highlighting the cleavage site (yellow arrow) relative to the consensus sequence (red) and anticodon (grey shaded). tRNAs were incubated with increasing amounts of VapC-mt4 (ratios of toxin to RNA were 0:1, 2.5:1 and 5:1) for 3 h at 37 °C. Convention when numbering tRNA bases dictates that the anticodon is designated as numbered positions 34–36. This convention is followed in b , d , f . Note, however, that for tRNA Ser26 ( d ) and tRNA Ser24 ( f ) the actual base numbers for the anticodon are 35–37. Complete gel images are shown in Supplementary Fig. 5 . 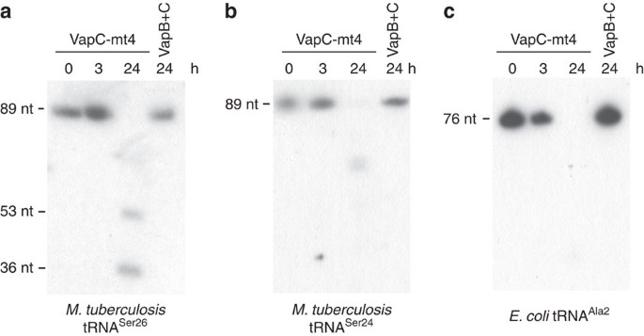Figure 4: VapC-mt4 also cleaves modifiedM. tuberculosistRNAs. (a,b) Total RNA (2 μg) was incubated with VapC-mt4 (20 pmol) for the times indicated, and northern analysis was performed using isoacceptor-specific oligonucleotides complementary to each ASL. VapB+C samples denote preincubation of the VapC-mt4 toxin (20 pmol) with VapB-mt4 antitoxin (120 pmol) before addition of total RNA. (c) Analogous experiment forE. colitRNAAla2usingE. colitotal RNA and an isoacceptor-specific oligonucleotide complementary to the ASL. Complete gel images are shown inSupplementary Fig. 6. Full size image Figure 4: VapC-mt4 also cleaves modified M. tuberculosis tRNAs. ( a , b ) Total RNA (2 μg) was incubated with VapC-mt4 (20 pmol) for the times indicated, and northern analysis was performed using isoacceptor-specific oligonucleotides complementary to each ASL. VapB+C samples denote preincubation of the VapC-mt4 toxin (20 pmol) with VapB-mt4 antitoxin (120 pmol) before addition of total RNA. ( c ) Analogous experiment for E. coli tRNA Ala2 using E. coli total RNA and an isoacceptor-specific oligonucleotide complementary to the ASL. Complete gel images are shown in Supplementary Fig. 6 . Full size image VapC-mt4 cleavage requires an ACGC in the proper context VapC-mt4 appears to require more than the consensus sequence alone since only tRNA Ala2 was cleaved even though there are 12 E. coli tRNAs containing a VapC-mt4 cleavage consensus sequence. Therefore, to better characterize the properties of RNA recognition and cleavage by this toxin, we first tested if VapC-mt4 cleavage at these consensus RNA sequences required single-stranded (ss) or double-stranded (ds) RNA. As with the MazF toxin [25] , VapC-mt4 also requires that the cleavage consensus sequence resides within ssRNA, since an RNA fragment containing the ACGC consensus sequence could only be cleaved as a ssRNA ( Fig. 5 , lanes 2,4). Increasing concentrations of a complementary RNA fragment (leading to the formation of dsRNA) resulted in a gradual decrease in cleavage ( Fig. 5 , lanes 4–9). 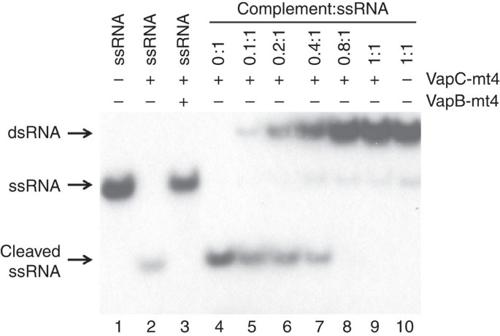Figure 5: VapC-mt4 cleavage requires a single-stranded RNA template. A 20-nt 5′ end-labelled RNA containing an ACGC consensus sequence alone (lane 1), after incubation with VapC-mt4 (lane 2), or after incubation; with VapB-mt4 and VapC-mt4 (lane 3). This 20-nt RNA was also preincubated with increasing amounts of an RNA complement lacking an ACGC consensus (lanes 4–10) followed by incubation with VapC-mt4. The positions of the dsRNA, ssRNA and cleaved ssRNA are shown on the left. The ratio of toxin to RNA was 64.2:1 and the assay was incubated at 37 °C for 3 h. A complete gel image is shown inSupplementary Fig. 7. Figure 5: VapC-mt4 cleavage requires a single-stranded RNA template. A 20-nt 5′ end-labelled RNA containing an ACGC consensus sequence alone (lane 1), after incubation with VapC-mt4 (lane 2), or after incubation; with VapB-mt4 and VapC-mt4 (lane 3). This 20-nt RNA was also preincubated with increasing amounts of an RNA complement lacking an ACGC consensus (lanes 4–10) followed by incubation with VapC-mt4. The positions of the dsRNA, ssRNA and cleaved ssRNA are shown on the left. The ratio of toxin to RNA was 64.2:1 and the assay was incubated at 37 °C for 3 h. A complete gel image is shown in Supplementary Fig. 7 . Full size image We next enlisted E. coli tRNA Asp3 as a tool to study the importance of context. tRNA Asp3 has the ACGC sequence located in the identical position as in E. coli tRNA Ala2 , yet VapC-mt4 only cleaved tRNA Ala2 ( Fig. 6 compare ‘wild-type’ tRNA red sequences). Interestingly, although these two tRNAs are 66% identical overall they differ at only three positions in their entire anticodon loop, two bases in the anticodon and one base just 5′ of the anticodon ( Fig. 6 compare sequences in ‘wild-type’ illustrations). To establish if the sequence of the anticodon influenced cleavage, we mutated the tRNA Ala2 anticodon to a GUC (the anticodon for tRNA Asp3 ) and the tRNA Asp3 anticodon to a UGC (the anticodon for tRNA Ala2 ; Fig. 6 ‘mutant’ panels). Wild-type tRNA Ala2 was efficiently cleaved, but the anticodon mutant version was no longer cleaved ( Fig. 6a ‘mutant’ panel). Conversely, tRNA Asp3 with a wild-type anticodon was not cleaved, while the mutated version was efficiently cleaved ( Fig. 6b ‘mutant’ panel). Therefore, the ACGC sequence is not the only determinant for RNA cleavage by VapC-mt4; the consensus sequence must be single-stranded and positioned in the tRNA such that all required conditions for proper recognition and cleavage are met. 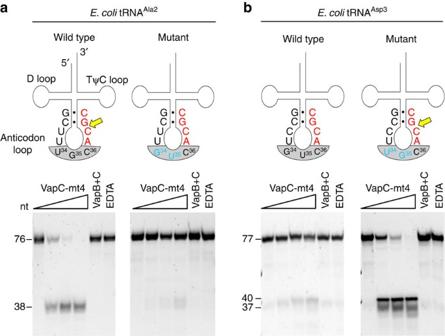Figure 6: VapC-mt4 cleavage requires an ACGC in the proper context. (a) Left panel, complete cleavage of wild-type tRNAAla2by VapC-mt4; right panel, no cleavage after mutation of two bases (blue) in the tRNAAla2anticodon to match those in tRNAAsp3. (b) Left panel, no cleavage of wild-type tRNAAsp3by VapC-mt4; right panel, complete cleavage after mutation of two bases (blue) in the tRNAAsp3anticodon to match those in tRNAAla2. Cleavage site (yellow arrow), consensus sequence (red), mutated bases (blue), anticodon (grey shaded), base pairing represented by black dots (·).In vitro-synthesized tRNAs were incubated with increasing amounts of VapC-mt4 (ratios of toxin to RNA were 0:1, 1.25:1, 2.5:1 and 5:1). Control reactions on the right contained the highest concentration of VapC-mt4 preincubated with VapB antitoxin or EDTA before addition of the respective tRNAs. Reactions were incubated at 37 °C for 3 h. Sizes of full-length and cleaved tRNA products on the left. The sizes of the tRNAAsp3mutant cleavage products are predicted based on the site of cleavage in tRNAAla2. Convention when numbering tRNA bases dictates that the anticodon bases are numbered 34–36. This convention is followed ina,b. Note, however, that in the case of tRNAAsp3(b) the actual base numbers for the anticodon are 35–37. Note that in some cases extra bands are visible for the cleavage products because the T7 RNA polymerase used to synthesize the tRNAs frequently leads to 3′ end heterogeneity (usually ±1 nt)61,62. Complete gel images are shown inSupplementary Fig. 8. Figure 6: VapC-mt4 cleavage requires an ACGC in the proper context. ( a ) Left panel, complete cleavage of wild-type tRNA Ala2 by VapC-mt4; right panel, no cleavage after mutation of two bases (blue) in the tRNA Ala2 anticodon to match those in tRNA Asp3 . ( b ) Left panel, no cleavage of wild-type tRNA Asp3 by VapC-mt4; right panel, complete cleavage after mutation of two bases (blue) in the tRNA Asp3 anticodon to match those in tRNA Ala2 . Cleavage site (yellow arrow), consensus sequence (red), mutated bases (blue), anticodon (grey shaded), base pairing represented by black dots (·). In vitro -synthesized tRNAs were incubated with increasing amounts of VapC-mt4 (ratios of toxin to RNA were 0:1, 1.25:1, 2.5:1 and 5:1). Control reactions on the right contained the highest concentration of VapC-mt4 preincubated with VapB antitoxin or EDTA before addition of the respective tRNAs. Reactions were incubated at 37 °C for 3 h. Sizes of full-length and cleaved tRNA products on the left. The sizes of the tRNA Asp3 mutant cleavage products are predicted based on the site of cleavage in tRNA Ala2 . Convention when numbering tRNA bases dictates that the anticodon bases are numbered 34–36. This convention is followed in a , b . Note, however, that in the case of tRNA Asp3 ( b ) the actual base numbers for the anticodon are 35–37. Note that in some cases extra bands are visible for the cleavage products because the T7 RNA polymerase used to synthesize the tRNAs frequently leads to 3′ end heterogeneity (usually ±1 nt) [61] , [62] . Complete gel images are shown in Supplementary Fig. 8 . Full size image VapC-mt4 recognizes sequence and structural determinants Having established that sequences in the anticodon immediately adjacent to a consensus sequence influence E. coli tRNA cleavage by VapC-mt4, we performed more detailed studies to further interrogate the importance of sequence and secondary structure elements within a biologically relevant subset of VapC-mt4 targets. We chose M. tuberculosis tRNA Ser24 from the three tRNAs cleaved by VapC-mt4 because it also contains an ACGC consensus site that bridges the junction between the anticodon stem and the anticodon loop, analogous to E. coli tRNA Ala2 ( Fig. 7 ). 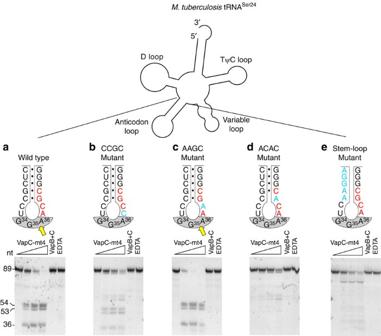Figure 7: tRNA cleavage by VapC-mt4 requires both structure and sequence determinants. (a–e) Secondary structure outline ofM. tuberculosistRNASer24(top) and cleavage assays comparing wild-type VapC-mt4 cleavage (a) with mutants that alter the consensus sequence but not ASL base pairing (b,c), a mutant that alters the consensus and disrupts one base pair in the stem (d), a mutant that retains the consensus sequence but removes all base pairing in the stem (e). Mutated bases (blue), cleavage site (yellow arrow), consensus sequence (red), anticodon (grey shaded), base pairing represented as black dots (·).In vitro-synthesized tRNAs were incubated with increasing amounts of VapC-mt4 (ratios of toxin to RNA were 0:1, 1.25:1, 2.5:1 and 5:1). Control reactions on the right contained the highest concentration of VapC-mt4 preincubated with VapB antitoxin or EDTA before addition of the respective tRNAs. Reactions were incubated at 37 °C for 3 h. Sizes of full-length and cleaved tRNA products on the left. Convention when numbering tRNA bases dictates that the anticodon bases are numbered 34–36. This convention is followed ina–e. Note however that in the case of tRNASer24(a–e) the actual base numbers for the anticodon are 35–37. Complete gel images are shown inSupplementary Fig. 9. Figure 7: tRNA cleavage by VapC-mt4 requires both structure and sequence determinants. ( a – e ) Secondary structure outline of M. tuberculosis tRNA Ser24 (top) and cleavage assays comparing wild-type VapC-mt4 cleavage ( a ) with mutants that alter the consensus sequence but not ASL base pairing ( b,c ), a mutant that alters the consensus and disrupts one base pair in the stem ( d ), a mutant that retains the consensus sequence but removes all base pairing in the stem ( e ). Mutated bases (blue), cleavage site (yellow arrow), consensus sequence (red), anticodon (grey shaded), base pairing represented as black dots (·). In vitro -synthesized tRNAs were incubated with increasing amounts of VapC-mt4 (ratios of toxin to RNA were 0:1, 1.25:1, 2.5:1 and 5:1). Control reactions on the right contained the highest concentration of VapC-mt4 preincubated with VapB antitoxin or EDTA before addition of the respective tRNAs. Reactions were incubated at 37 °C for 3 h. Sizes of full-length and cleaved tRNA products on the left. Convention when numbering tRNA bases dictates that the anticodon bases are numbered 34–36. This convention is followed in a – e . Note however that in the case of tRNA Ser24 ( a – e ) the actual base numbers for the anticodon are 35–37. Complete gel images are shown in Supplementary Fig. 9 . Full size image We had previously determined that the GC residues in the ACGC recognition sequence are essential for VapC-mt4 cleavage of a synthetic 20-nt RNA template [19] . To test the importance of the first two AC residues, we mutated each individually, incubated with VapC-mt4, and assessed the extent of cleavage ( Fig. 7a–c ). First, we synthesized tRNA Ser24 with the first A in the ACGC sequence mutated to a C. In comparison with the complete cleavage of wild-type tRNA Ser24 using the highest concentration (10 pmol) of VapC-mt4, an ACGC→ C CGC mutant was cleaved less efficiently ( Fig. 7a,b ). Second, we synthesized an ACGC→A A GC mutant and found that it was cleaved as efficiently as wild type ( Fig. 7c ). Third, we altered the ACGC consensus sequence to create minor or major changes in secondary or tertiary structure of the ASL. An ACGC→AC A C mutation, now lacking the G–C base pair at the stem of the ASL as well as one of the two critical consensus residues, severely impaired cleavage ( Fig. 7d ). Therefore, three of the four bases in the VapC-mt4 ACGC cleavage consensus sequence are important for cleavage. Cleavage was less efficient when the first A of the consensus was mutated, and mutation of the G or terminal C (previously reported by Sharp et al. [19] ) abolished cleavage. Finally, introducing mutations in the ASL that disrupt base pairing while keeping the ACGC consensus intact, yielded a marginal level of cleavage but at a different position ( Fig. 7e ). We conclude that recognition of specific tRNA targets by VapC-mt4 requires proper sequence and structural context. Simulated docking of VapC-mt4 and tRNA Interestingly, in contrast to E. coli tRNA Ala2 (whose cut site is A 37 C 38 ↓G 39 C 40 ), the cleavage sites for each of the three M. tuberculosis tRNAs are in proximity to, but not within their consensus sequences. To model how VapC-mt4 may potentially interact in distinct ways with either tRNA Ala2 or tRNA Ser24/6 , we performed protein–RNA docking simulations using the programme 3dRPC [26] ( Fig. 8 ). Since a structure of VapC-mt4 has not been determined, we generated a homology model of VapC-mt4 using the HHpred homology model workflow and Modeller [27] , [28] from three published structures: M. tuberculosis VapBC5 (PDB accession code 3DBO [29] ), Rickettsia VapBC2 (PDB accession code 3ZVK [30] ) and FitAB (PDB accession code 2H1C [31] ). On the basis of the published stoichiometry of VapC homologues [32] , [33] , a VapC-mt4 dimer was generated through simulated docking using GRAMM-X [27] , [34] and then the interactions between the complex were optimized with RosettaDock [35] . There are also no structures for any of the three VapC-mt4 targets. But tRNA Phe and tRNA Leu (PDB accession codes 4TNA, chain A and 3UZ3, chain B [36] ) are close homologues of tRNA Ala2 and tRNA Ser24/6 , respectively. We used tRNA Leu as a representative for both serine isotypes recognized by VapC-mt4 as they all contain an expanded variable loop. The position of a divalent cation in our model was extrapolated by superpositioning the structure of Pyrobaculum aerophilum VapC with a coordinated divalent cation with our VapC-mt4 model generated by DaliLite (PDB accession code 2FE1 (ref. 32 )) [38] . On the basis of the alignment we predict that VapC-mt4 residues Asn98 and Asn116 likely coordinate a metal ion in its active site due to the proximity of the P. aerophilum VapC equivalent. 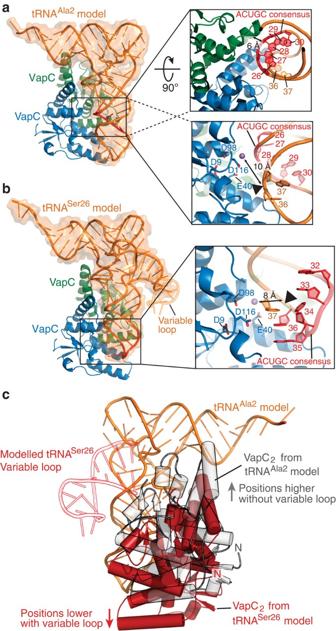Figure 8: VapC-mt4-tRNA docking simulations. (a) Predicted binding of a (VapC-mt4)2(blue and green) to tRNAAla2(Type I tRNA homologue, tRNAPhemodel shown in orange; PDB accession code 4TNA) using a protein–RNA docking simulation programme 3dRPC. The consensus sequence 5′-ACUGC-3′ is highlighted in red and boxed. The upper right boxed magnification shows a 90° rotated view highlighting the proximity of the tRNA consensus sequence to the VapC monomer not thought to be involved in activity (green). The lower right boxed magnification is a detailed view of the cleavage site. The VapC-mt4 key residues, tRNA consensus sequence and the target nucleotides are shown as sticks, with a black triangle indicating the cleavage site. (b) Predicted binding of a (VapC-mt4)2(blue and green) to tRNASer24/Ser26(Type II tRNA homologue, tRNALeumodel shown in orange; PDB accession code 3UZ3). The expanded variable loop of tRNASer26is depicted in orange outline and the consensus sequence 5′-ACUGC-3′ is highlighted in red. The boxed magnification is a detailed view of the cleavage site showing the VapC-mt4 key residues, the tRNALeuconsensus sequence and the target nucleotides are shown in sticks, with a black triangle indicating the cleavage site. The extrapolated position of a divalent cation is shown as a purple sphere in botha,b. (c) A comparison of (VapC-mt4)2binding, highlighting the positional shift in tRNA binding depending on the target tRNA type (grey, tRNAAla2; red, tRNASer24/Ser26). The presence of expanded variable loop in tRNASer26(shown in red outline) influences the binding of VapC-mt4 (positions lower in anticodon loop) possibly explaining the difference observed in target cleavage sites. Convention when numbering tRNA bases dictates that the anticodon bases are numbered 34–36. This convention is followed ina–c. Note however that in the case of tRNASer26/Ser24(b,c) the actual base numbers for the anticodon are 35–37. Figure 8: VapC-mt4-tRNA docking simulations. ( a ) Predicted binding of a (VapC-mt4) 2 (blue and green) to tRNA Ala2 (Type I tRNA homologue, tRNA Phe model shown in orange; PDB accession code 4TNA) using a protein–RNA docking simulation programme 3dRPC. The consensus sequence 5′-ACUGC-3′ is highlighted in red and boxed. The upper right boxed magnification shows a 90° rotated view highlighting the proximity of the tRNA consensus sequence to the VapC monomer not thought to be involved in activity (green). The lower right boxed magnification is a detailed view of the cleavage site. The VapC-mt4 key residues, tRNA consensus sequence and the target nucleotides are shown as sticks, with a black triangle indicating the cleavage site. ( b ) Predicted binding of a (VapC-mt4) 2 (blue and green) to tRNA Ser24/Ser26 (Type II tRNA homologue, tRNA Leu model shown in orange; PDB accession code 3UZ3). The expanded variable loop of tRNA Ser26 is depicted in orange outline and the consensus sequence 5′-ACUGC-3′ is highlighted in red. The boxed magnification is a detailed view of the cleavage site showing the VapC-mt4 key residues, the tRNA Leu consensus sequence and the target nucleotides are shown in sticks, with a black triangle indicating the cleavage site. The extrapolated position of a divalent cation is shown as a purple sphere in both a , b . ( c ) A comparison of (VapC-mt4) 2 binding, highlighting the positional shift in tRNA binding depending on the target tRNA type (grey, tRNA Ala2 ; red, tRNA Ser24/Ser26 ). The presence of expanded variable loop in tRNA Ser26 (shown in red outline) influences the binding of VapC-mt4 (positions lower in anticodon loop) possibly explaining the difference observed in target cleavage sites. Convention when numbering tRNA bases dictates that the anticodon bases are numbered 34–36. This convention is followed in a – c . Note however that in the case of tRNA Ser26/Ser24 ( b , c ) the actual base numbers for the anticodon are 35–37. Full size image While both docked models indicate that one active site from each VapC-mt4 dimer is positioned adjacent to the experimentally determined tRNA cleavage site located in the anticodon loop, the overall (VapC-mt4) 2 orientations differ depending on the tRNA it recognizes. In the VapC-mt4 dimer-tRNA Phe/Ala2 model, one monomer of VapC-mt4 is predicted to interact with the base paired anticodon stem of the tRNA with potential additional contacts with the D loop ( Fig. 8a ). The other monomer of VapC and its active site is modelled adjacent to the predicted cleavage site between residues 36 and 37 ( Fig. 8a , right panel). However in the VapC-mt4 dimer-tRNA Leu/Ser26 model, the large expanded variable loop likely causes the protein/toxin to recognize the anticodon stem closer toward the anticodon ( Fig. 8b ). Large expanded variable loops are present in both tRNA Leu and tRNA Ser ; therefore, we predict this influences the location of the cleavage site. Also in this case, the active site in one VapC monomer is positioned adjacent to the tRNA backbone near cleavage site residue 36 ( Fig. 8b , right panel). Interestingly, the tRNA Ala model shows significant interactions with the 5′-ACUGC-3′ consensus sequence in contrast to the tRNA Ser model, which shows minimal interactions ( Fig. 8c ). VapBC modules are among the most prevalent TA systems in the genomes of a variety of pathogens, comprising >40% of the ∼ 700 TA modules identified in 126 complete genomes of free-living bacteria [39] . Therefore, when organisms carry multiple members of a TA system family, VapBC systems are inexplicably the most abundant. The multiple iterations of VapBC TA systems (though none are identical) are associated with increased virulence in the pathogens that contain them, accounting for the origin of the name Vap, for virulence-associated protein [40] . A detailed understanding of the properties of M. tuberculosis VapC paralogs is essential for interpretation of their physiological role in M. tuberculosis and other pathogens. We studied a representative family member, M. tuberculosis VapC-mt4 (aka VapC4), to obtain a better understanding of the RNA targets and molecular mechanism of VapC toxin recognition and cleavage. In contrast to VapC-mt20, which cleaves 23S rRNA at the sarcin–ricin loop [20] , VapC-mt4 specifically targeted just three of the 45 total M. tuberculosis tRNA isotypes—tRNA Ala2 , tRNA Ser26 and tRNA Ser24 . All three of these tRNAs contain one of the cleavage consensus sequences for this toxin identified in our earlier report, namely ACGC or ACUGC. Two tRNAs contained the ACUGC recognition sequence, which was the strongest cleavage site among 12 sites in the ∼ 3.5-kb bacteriophage MS2 RNA template that were cut by VapC-mt4 (ref. 19 ). Thus, cleavage of tRNA involves sequence recognition by VapC-mt4. This contrasts with 23S rRNA cleavage by VapC-mt20, which appears to be more dependent on recognition of the stem loop structure of the sarcin–ricin loop [20] . In fact, VapC-mt4 differs from all other TA system toxins, the majority of which (1) predominantly cleave mRNA independent of the ribosome and at all cleavage consensus sequences (MazF family) or (2) cleave mRNA in a ribosome-dependent manner with no clear sequence specificity (RelE family) or some degree of sequence specificity (HigB, YafQ toxins). Tertiary fold or recognition of determinants in the sugar-phosphate backbone appears to also contribute to the selectivity of VapC-mt4, given that many other M. tuberculosis tRNAs also harbor the same recognition sequence yet only a few are efficiently cleaved. While tRNAs generally adopt L-shaped three-dimensional structures to enable entry into the ribosome, there may be some subtle variation in the overall structure that can be distinguished by VapC-mt4. In fact, while all tRNAs possess three stem-loops (D, anticodon, TΨC), the cloverleaf secondary structures of tRNA do vary slightly. Type II tRNAs (tRNA Ser26 and tRNA Ser24 in our case) also contain an extended variable arm between the anticodon and TΨC stem loop ( Fig. 3 ). Also, although the D arm usually has a 4-bp stem, tRNA Ser26 and tRNA Ser24 , have a 3-bp stem. In fact, our simulated docking experiments indicate that the variable loop influences the positioning of the VapC-mt4 dimer on the tRNA, which we propose alters the location of the cleavage site ( Fig. 6 ). Independent of tertiary fold, the interaction of VapC-mt4 with the sugar-phosphate backbone may contribute to cleavage specificity. On the basis of studies of tRNA recognition for aminoacylation of tRNA Gln by glutaminyl-tRNA synthetase, class II tRNA synthetase interaction with the sugar-phosphate backbone is an important recognition determinant in addition to base recognition at the anticodon loop, at the acceptor end, and with the interior base pair of the D stem [41] . Strikingly, VapC-mt4 cuts all three M. tuberculosis tRNA targets precisely within the anticodon loop. In the case of tRNA Ala2 , VapC-mt4 cleaves at the position immediately 3′ adjacent to the anticodon ( Fig. 3b ). For tRNA Ser26/4 , VapC-mt4 cleavage occurs within the anticodon itself between the second and the third nucleotides ( Fig. 3d,f ). However, there was no correlation between the tRNA isoacceptors targeted for cleavage and their corresponding codon usage preferences. tRNA Ala2 decodes the lowest percentage of alanine codons (10%) in M. tuberculosis , while tRNA Ser26 (26%) and tRNA Ser24 (21%) decode intermediate percentages of serine codons (with tRNA Ser28 decoding the highest number of serine codons, 35%). Since the ASL of tRNA interacts with the decoding centre of the 30S subunit, cleavage at the anticodon sequence of the ASL by VapC-mt4 is consistent with the known inhibition of translation by VapC-mt4 on overexpression in E. coli using an arabinose-inducible plasmid (<10% of wild type [19] ). In some strains of E. coli , colicins are secreted into the environment to kill the neighbouring bacterial cells and reduce competition [42] . Colicins D and E5 enlist cleavage of tRNA at a single site within the ASL to inhibit translation and cause cell death. The lethality of colicin D is due to specific cleavage of all four tRNA Arg isoacceptors between positions 38 and 39, corresponding to the junction of the loop and stem on the 3′ side of the anticodon [43] . Likewise, Salmonella/Shigella VapC cleaves tRNA fMet at the same position as colicin D [16] . As with VapC-mt4, colicin E5 cleaves within the anticodon loop, at positions 34 and 35 of the anticodon [44] . Also serving a defensive role, the E. coli endoribonuclease PrrC triggers cell suicide by cleaving tRNA Lys between anticodon positions 33 and 34 in response to bacteriophage T4 infection of E. coli cells [45] , [46] , [47] . Therefore, colicins D, E5 and PrrC all cause cell death. In the case of colicins D and E5, death is undoubtedly due to the absence of their cognate immunity proteins in neighbouring cells that take up the colicins alone [42] , [43] . For PrrC-mediated cell death, it is thought that after T4 phage infection, the Stp phage protein alters the association of the ‘antitoxin’ Eco prrI with PrrC, releasing free PrrC and leading to unchecked cleavage of lysine tRNA [45] , [46] , [47] . In contrast, the general physiological role of most TA systems, including VapC-mt4, appears to involve stress survival and not cell death due to the presence of a cognate antitoxin that dynamically regulates toxin activity in response to stress [3] . In fact, as demonstrated for the MazF toxin, cell death can be precluded following toxin activation when the cognate antitoxin is also expressed [2] . Cell death only occurs after prolonged activation of the toxin, when the cell reaches ‘the point of no return’ [2] . Our earlier study showed that VapC-mt4 overexpression results in translation inhibition with accumulation of polysomes, indicative of a block at the elongation step [19] . Possibly, ribosomal stalling may result from a non-productive interaction of the cleaved ASL with the A site of the ribosome. In addition, two studies have demonstrated that cleavage or alteration of the ASL leads to defects in aminoacylation. First, a break in the phosphodiester backbone of the ASL between position 34 and 35 of yeast tRNA Met inhibits aminoacylation [48] . Second, aminoacylation by E. coli glutaminyl-tRNA synthetase requires recognition of the sugar-phosphate backbone at positions 34–38 (ref. 41 ). Therefore, disruption of the backbone by cleavage between position 36 and 37 by VapC-mt4 would also likely disrupt aminoacylation by class II synthetases, potentiating its effect on translation and growth. VapC-mt4 targets a small subset of M. tuberculosis tRNAs with exquisite specificity. It not only distinguishes between tRNA isotypes, it selectively cleaves some, but not all, isoacceptors. More specifically, VapC-mt4 cleaves one isoacceptor of tRNA Ala (tRNA Ala2 ) of the three represented in M. tuberculosis and two of the four isoacceptors of tRNA Ser (tRNA Ser26 and tRNA Ser24 ) are cleaved efficiently. Although colicins D and E5 exhibit specificity for tRNAs, their tRNA targets are either limited to all four tRNA Arg isoacceptors (colicin D [43] ) or extend to four isotypes (tRNA Asn , tRNA Asp , tRNA Tyr and tRNA His for colicin E5 (ref. 44 )). Since our data identifies the presence of the cleavage consensus sequence ACGC or ACUGC as one major determinant for tRNA cleavage, some of the selectively of VapC-mt4 is attributed to this requirement since not all isoacceptors of tRNA Ser harbour this essential sequence. In contrast, the sequence requirements for colicins appear to be less specific than for VapC-mt4—colicin E5 cleaves at (C/T)GU [49] , while the interrogation of sequence requirements for colicin D has not been reported [43] . No atomic level structures of colicins bound to tRNAs have been reported. Structural studies of VapC-mt4 bound to tRNA will be instrumental in pinpointing additional determinants (tertiary fold and/or sugar-phosphate backbone interactions) that guide toxin specificity for a handful of tRNA targets. Although the precise physiological triggers for VapC-mt4 have not yet been identified, we know that the expression of this toxin leads to growth inhibition in M. tuberculosis [14] , [19] . In fact, with few exceptions, the unifying feature of TA systems is their role as stress responsive growth regulators. Consistent with this role, there is mounting evidence linking increased expression of TA systems with several stresses in M. tuberculosis , especially those encountered during latent tuberculosis [4] , [5] , [6] , [7] , [8] , [9] , [10] , [11] , [12] , [13] . As a complement to transcript-oriented studies, recent proteomic profiles generated from parallel analyses by mass spectrometry and two-dimensional differential gel electrophoresis reinforced the role of TA systems in stress [50] . Culture filtrates from M. tuberculosis cells after nutrient starvation contained elevated levels of 13 TA toxins, including a >10-fold increase in VapC-mt4 (ref. 50 ). The need for the high number of VapC toxins in M. tuberculosis (48 predicted) is not yet clear. All VapC toxins are expected to function as nucleases due to the presence of a PIN domain. However, our findings reported here coupled with those of the only other well-characterized M. tuberculosis VapC toxin—VapC20, which targets the 23S rRNA sarcin–ricin loop [20] —suggest that the VapC family members will not be functionally redundant. Instead, each VapC may cleave unique substrates or sites within a given target, thus allowing a defined molecular response to one or more stresses. Given that M. tuberculosis cells can remain dormant yet viable for many years in latent tuberculosis in a granuloma, the resulting activity of each toxin may impart some degree of growth downregulation that is then lifted before cells reach the point of no return. Thus, through activation of a shifting array of VapC toxins in a calibrated, asynchronous manner, M. tuberculosis may be able to limit growth while never reaching the point of cell death. Interestingly, the presence of cleaved tRNA halves and smaller fragments is also emerging as a hallmark of stress responses in many eukaryotes (reviewed in refs 51 , 52 , 53 ). In this rapidly evolving area, tRNA halves or other tRNA-derived fragments have been associated with a range of functions, including translational control, apoptosis and RNA interference regulation. Therefore, our results uncover a new parallel between the VapC-mt4 toxin-mediated stress response in M. tuberculosis and post-transcriptional tRNA cleavage at the ASL during stress in eukaryotes. Since the activities of only two VapC toxins have been characterized, it is highly likely that more VapC toxins will also target tRNAs. This would further expand the repertoire of tRNAs acting in a non-conventional role, shed light on the conundrum of why M. tuberculosis cells have so many VapBC TA systems and strengthen our understanding of how their orchestrated expression impacts stress survival, growth and virulence. Strains and plasmids The E. coli strain BL21(DE3) (F- omp T hsd S β (r β -m β ) dcm gal (DE3) tonA) (Novagen) was used for protein expression. The E. coli strain BW25113Δ6 (F − lacI q rrnB T14 Δ lacZ WJ16 hsdR514 Δ araBAD AH33 Δ rhaBAD LD78 Δ mazEF Δ chpBIK Δ relBE Δ yefM-yoeB Δ dinJ-yafQ ) [21] was used for the isolation of RNA. E. coli K-12 Mach1 T1 cells (Δ rec A1398 end A1 ton A Φ80Δ lac M15 Δ lac X74 hsd R(r k + m k + ); Invitrogen) were used for all cloning experiments. The pBAD33-VapC-mt4 and pET28a-His 6 -VapC-mt4 was described in our earlier work [19] . All E. coli liquid cultures were grown in M9 minimal media supplemented with 0.2% (w/v) casamino acids, 1 mM MgSO 4 , 0.001% (w/v) thiamine and either 0.2% glucose or 0.2% glycerol at 37 °C. 1 mM isopropyl 1-thio-β- D -galactopyranoside, 0.2% arabinose, 45 μg ml −1 kanamycin and 25 μg ml −1 chloramphenicol were added to culture medium as required. Purification of recombinant VapC-mt4-His 6 E. coli BL21(DE3)pLysE was transformed with the pET28a-His 6 -VapC-mt4 plasmid. Transformants were selected and grown in 1 l of M9 minimal media containing 0.2% glucose at 37 °C to an OD 600 of 0.6–0.8 and toxin expression induced with isopropyl 1-thio-β- D -galactopyranoside for 4 h. Recombinant VapC-mt4 was then purified as previously described [19] . In brief, the cells were lysed by sonication. Cell lysates were centrifuged at 32,000 g for 10 min to remove cell debris. Protein was then purified from the cleared cell lysates by nickel–nitrilotriacetic acid affinity chromatography (Qiagen). Double-stranded RNA cleavage A 20-base ACGC-containing RNA oligonucleotide, NWO1430 (5′-AGGAAGAUACGCGAUAUGAA-3′), was 5′ end labelled with [γ- 32 P]-ATP using T4 polynucleotide kinase (NEB) following the manufacturer’s protocol. The labelled oligonucleotide was diluted with diethylpyrocarbonate (DEPC) -treated water to yield a final concentration of 0.2 pmol μl −1 . The labelled RNA was then mixed with different amounts (at ratios of 0:1, 0.1:1, 0.2:1, 0.4:1, 0.8:1 and 1:1) of a complementary RNA oligo, NWO1541 (5′-UUCAUAUCGCGUAUCUUCCU-3′). The two oligonucleotides were incubated at 70 °C for 3 min and then allowed to cool slowly to room temperature ( ∼ 30 min). Samples were adjusted to 10 mM Tris pH 7.5, 150 mM NaCl, 10 mM MgCl 2 ; 20 units of RNase inhibitor (NEB) was then added to each reaction followed by 17 pmol of VapC-mt4 (when indicated) in a final volume of 10 μl. The samples were incubated at 37 °C for 1 h and reactions stopped by adding 10 μl of sequence loading buffer (95% formamide, 20 mM EDTA, 0.05% bromophenol blue, 0.05% xylene cyanol FF). Samples were then heated to 95 °C for 5 min before electrophoresis on a 15% polyacrylamide, 7 M urea gel. In vitro synthesis of tRNA E. coli and M. tuberculosis tRNAs were synthesized in vitro following the method described by Sisido et al. [54] with minor modifications. In brief, a synthetic DNA oligonucleotide containing the T7 RNA polymerase promoter and the 5′ end of the tRNA gene of interest was annealed to a second oligonucleotide corresponding to the 3′ end of the tRNA gene. The annealed oligonucleotides were then extended using Taq DNA polymerase to create dsDNA containing the entire tRNA gene preceded by the T7 promoter. The product was then resolved on a 2% agarose gel to confirm its size and purified using the QIAquick Gel Extraction Kit (Qiagen). The sequence of the product was verified by automated DNA sequence analysis. Two-hundred ng of the tRNA gene was then transcribed in vitro using the RiboMAX Large Scale RNA Production System (Promega) as recommended by the manufacturer. The transcription reaction was separated on a 9% polyacrylamide, 7 M urea gel and visualized by staining with EtBr to confirm the size and purity of the transcribed tRNA. The tRNA transcript was then excised from the gel and incubated for 18 h at 37 °C in elution buffer (1 mM EDTA, 0.5 M ammonium acetate, 10 mM magnesium acetate, 0.1% SDS). The eluate was then collected, and the gel pieces were washed in fresh elution buffer. The elution and wash were combined, the tRNA was ethanol precipitated and resuspended in nuclease-free water. Purification of tRNA from E. coli cell extracts Total E. coli RNA was isolated using the hot phenol method. A culture of E. coli BW25113Δ6 was grown in M9 medium until the OD 600 reached a value of ∼ 0.6. The cells were pelleted and resuspended in 500 μl Buffer A (0.5% SDS, 20 mM sodium acetate, pH 4.0; 10 mM EDTA) and 500 μl phenol, pH 4.0. After vortexing to completely resuspend the cell pellet, the samples were heated to 60 °C for 10 min and centrifuged to separate the phases. The RNA-containing aqueous phase was removed, ethanol precipitated and resuspended in nuclease-free water. Individual tRNAs were then isolated from the total RNA using a biotinylated oligonucleotide that specifically annealed to tRNA Ala2 adapted from the procedure of Yokogawa et al. [55] . We first washed 450 μl of MagneSphere magnetic beads (Promega) three times (we used a magnetic stand to recover the beads after all wash and hybridization steps) with 600 μl of wash buffer (10 mM Tris-HCl pH 7.5, 1 mM EDTA and 1 M NaCl). We then added 600 pmol of the 5′ biotinylated oligonucleotide for tRNA Ala2 isolation, NWO1974 (5′-Biotin-AGACCTCCTGCGTGCAAAGCAGGC-3′), adjusted the volume to 300 μl with 10 mM Tris-HCl pH 7.5 and incubated at room temperature for 15 min with gentle inversion every 3 min. After binding of the tRNA Ala2 -specific oligonucleotide, the beads were washed three times with wash buffer. After the final wash, the beads were resuspended in 50 μl hybridization buffer (20 mM Tris-HCl pH 7.6, 1.8 M tetramethylammonium chloride (TMA-Cl), 0.2 mM EDTA). One mg of total RNA in 50 μl nuclease-free water was then added to the beads. Samples were then gently inverted, heated to 65 °C for 3 min and placed at 60 °C for 20 min with inversion every 4 min. The supernate containing unbound RNA was separated from the beads and transferred to a fresh tube and saved for rebinding. The beads containing the bound tRNAs were washed six times with 800 μl Tris-HCl, pH 7.6. The target tRNA was then eluted from the beads with 150 μl of Tris-HCl, pH 7.6 heated to 75 °C for 5 min and transferred to another tube containing 2 μl of 1 M MgCl 2 to assist in proper folding. To maximize recovery of tRNA, we repeated the last step with the saved aliquot and combined elutions. In vitro tRNA cleavage Cleavage of tRNAs produced via T7 transcription or purified from total RNA was performed in vitro following the assay described by Winther and Gerdes [16] with slight modifications. In brief, 2 pmol of tRNA was incubated with 2.5, 5 or 10 pmol of VapC-mt4 at 37 °C for 3 h in 10 mM HEPES pH 7.5, 15 mM KCl, 3 mM MgCl 2 , 10% glycerol in a final volume of 10 μl. To check for cleavage inhibition by the cognate antitoxin, VapB-mt4 was preincubated with VapC-mt4 for 15 min at 37 °C before the RNA substrate was added. In samples containing EDTA, 1 μl of 125 mM EDTA was added to the reaction before the addition of the RNA substrate. The products of these reactions were separated on a 9% polyacrylamide, 7 M urea gel and visualized by SYBR Gold (Invitrogen) staining. In vivo primer extension E. coli BW25113Δ6 cells carrying pBAD33-VapC-mt4 were grown in M9 minimal media containing 0.2% glycerol at 37 °C to an OD 600 of 0.3–0.4. Arabinose was then added to a final concentration of 0.2%. Aliquots were removed 0, 20, 40, 60, 80 and 100 min post induction and total RNA was extracted as described in the ‘Purification of tRNA from E. coli cell extracts’ section above. The primer NWO1976 (5′-GGGATCGAACCGCAGACC-3′) was 5′ end labelled with [γ- 32 P]ATP using T4 polynucleotide kinase (NEB). Five μg of total RNA was mixed with 40 pmol of the labelled oligonucleotide in a 6.5-μl reaction containing annealing buffer for the SuperScript III reverse transcriptase (Invitrogen). The samples were heated to 80 °C for 3 min and allowed to cool slowly to room temperature over 30 min. First Strand Reaction Mix (3.5 μl; Invitrogen) and 2 μl SuperScript III Enzyme Mix (Invitrogen) were then added. The reactions were incubated at 52 °C for 90 min, then heat inactivated at 70 °C for 10 min followed by addition of 12 μl of sequence loading buffer (95% formamide, 20 mM EDTA, 0.05% bromophenol blue and 0.05% xylene cyanol). The DNA-sequencing ladders for primer extension reactions were prepared using the Sequenase Version 2.0 DNA-Sequencing Kit (Agilent) as recommended. In vitro primer extension T7-transcribed M. tuberculosis tRNAs were cleaved as described in the ‘ In vitro tRNA cleavage’ section, purified by phenol:chloroform extraction and ethanol precipitated. Primer extension reactions were then performed as described in the previous section using 2 pmol of cleaved tRNA. Primers: tRNA Ala2 , NWO2164 (5′-GGAGCCTAGGGGACTCGAA-3′); tRNA Ser26 , NWO2165 (5′-GAGGCGAGAGGATTTGAACCTCC-3′); and tRNA Ser24 , NWO2166 (5′-GGAGGATGCGGGATTTGAACCC-3′). RNA-seq of E. coli RNA E. coli BW25113Δ6 cells carrying pBAD33-VapC-mt4 were grown in M9 minimal media containing 0.2% glycerol at 37 °C to OD 600 0.3–0.4. The culture was split in half and arabinose was then added to a final concentration of 0.2% to one of the cultures. Aliquots from induced and uninduced cultures were removed 0, 20, 40, 60, 80 and 100 min post induction. Total RNA was extracted as described in the ‘Purification of tRNA from E. coli cell extracts’; 5′ RNA-seq was performed using total RNA from the 20-min induced and uninduced cultures. The 20-min induction time was selected because it coincided with the initiation of toxicity, ensuring that the cleavage site being documented was the direct consequence of toxin induction and not due to secondary effects. Two pools of RNA, those possessing a 5′-P and those possessing a 5′-OH. After removal of 5′-P RNA from the 5′-OH pool, the resulting 5′-OH RNA was converted to 5′-P RNA via phosphorylation by 50 U OptiKinase. A 5′ SOLiD RNA adaptor was then ligated onto RNA from both pools. Reverse transcription and PCR was then performed based on the methods outlined in Schifano et al. [21] and Vvedenskaya et al. [56] . tRNA northern analysis Total RNA was isolated from E. coli as described above. Total RNA from M. tuberculosis H37Rv was isolated as previously described [57] . In brief, M. tuberculosis cells were grown to exponential phase and then pelleted. Cell pellets were resuspended in TRIzol Reagent (Invitrogen). RNA was treated with TURBO DNase (Invitrogen). Total RNA (2 μg) from each organism was incubated with 20 pmol of VapC-mt4 in a 10-μl reaction containing 10 mM HEPES pH 7.5, 15 mM KCl, 3 mM MgCl 2 , 10% glycerol at 37 °C for 0, 3 or 24 h. To check for cleavage inhibition by the cognate antitoxin, 120 pmol VapB-mt4 was preincubated with VapC-mt4 for 15 min at 37 °C before the RNA substrate was added and incubated at 37 °C for 24 h. The products of these reactions were separated on a 9% polyacrylamide, 7 M urea gel and visualized by SYBR Gold (Invitrogen) staining. RNA was transferred to nitrocellulose and hybridized with oligonucleotides specific for a given tRNA species. The oligonucleotides used were: E. coli tRNA Ala2 , NWO2268, 5′-CGTGCAAAGCAGGCGCTC-3′; M. tuberculosis tRNA Ser26 , NWO2277, 5′-GCAGTGAGCCCCATTCG-3′; and M. tuberculosis tRNA Ser24 , NWO2270, 5′-CCCTTGAAGGGGGACAACTCATTA-3′. VapC-mt4-tRNA molecular modelling All protein–RNA docking simulations were performed with the programme 3dRPC [26] . The homology model of VapC-mt4 was generated by the HHpred homology model workflow and Modeller using the optimal multiple template function [27] , [28] . The structural templates used in Modeller to generate the VapC-mt4 homology model were Rickettsia felis VapC (from VapBC2 complex; PDB accession code 3ZVK, chain A [30] ; 19% identity, 28.7% similarity to VapC-mt4), M. tuberculosis VapC (from VapBC5 complex; PDB accession code 3DBO, chain B [29] ; 36% identity, 53.7% similarity) and Neisseria gonorrhoeae FitB (from FitAB complex; PDB accession code 2H1C, chain A [31] ; 27% identity, 28.8% similarity). The VapC-mt4 homology dimer models were first generated by the global search programme GRAMM-X [27] , [34] , followed by further refinement using the programme RosettaDock [35] . The manganese atom was positioned in the VapC-mt4 homology model using an alignment of Pyrobaculum aerophilum VapC (PDB accession code 2FE1) [32] generated by DaliLite [38] . The homologue of tRNA Ala2 used in this study was Saccharomyces cerevisiae tRNA Phe (PDB accession code 4TNA, chain A) [37] and the homologue for the tRNA Ser26 was Escherichia coli tRNA Leu (PDB accession code 3UZ3, chain B) [36] . The expanded variable loop of M. tuberculosis tRNA Ser26 was generated by the programme 3dRNA using the secondary structure predicted by NAVIEW [58] , [59] and extrapolated onto the tRNA Leu variable loop by least-squares fitting using Coot [60] . With both tRNA models, the changes in the target anticodon loop residues corresponding to tRNA Ala2 or tRNA Ser26 sequences were manually introduced using Coot. The proposed models were selected based on the proximity between the targeted region of the tRNA ASL and the proposed VapC catalytic residues. Accession codes : The RNA sequencing data have been deposited in the NCBI Sequence Read Archive under accession code PRJNA277981 . How to cite this article : Cruz, J.W. et al. Growth-regulating Mycobacterium tuberculosis VapC-mt4 toxin is an isoacceptor-specific tRNase. Nat. Commun. 6:7480 doi: 10.1038/ncomms8480 (2015).